Two susceptibility loci identified for prostate cancer aggressiveness Most men diagnosed with prostate cancer will experience indolent disease; hence, discovering genetic variants that distinguish aggressive from nonaggressive prostate cancer is of critical clinical importance for disease prevention and treatment. In a multistage, case-only genome-wide association study of 12,518 prostate cancer cases, we identify two loci associated with Gleason score, a pathological measure of disease aggressiveness: rs35148638 at 5q14.3 ( RASA1 , P =6.49 × 10 −9 ) and rs78943174 at 3q26.31 ( NAALADL2 , P =4.18 × 10 −8 ). In a stratified case–control analysis, the SNP at 5q14.3 appears specific for aggressive prostate cancer ( P =8.85 × 10 −5 ) with no association for nonaggressive prostate cancer compared with controls ( P =0.57). The proximity of these loci to genes involved in vascular disease suggests potential biological mechanisms worthy of further investigation. Prostate cancer is the most common cancer diagnosed in men and second leading cause of cancer death among men in the United States [1] ; however, little is known about why the disease progresses in some men but not in others. Determining which cancers are likely to progress and cause death is of critical clinical importance. Prostate cancer aggressiveness is thought to be partially determined by genetic factors, as studies have shown an increased risk of death from prostate cancer among offspring with a family history of fatal disease [2] , [3] . The definitions of aggressive prostate cancer differ between studies; however, one important and widely used descriptor is tumour grade at diagnosis, as measured by the Gleason score, which ranks pathological changes, namely, tumour differentiation, and has been associated with disease progression and survival [4] . Linkage studies using the Gleason score as a measure of aggressiveness have implicated several chromosomal regions, including 1p, 5q, 6q, 7q and 19q; however, no specific genetic mutations have been conclusively identified [5] , [6] , [7] , [8] . Although previous genetic association studies have identified or suggested markers for aggressive prostate cancer [9] , [10] , [11] , these single-nucleotide polymorphisms (SNPs) have either also been associated with nonaggressive disease, making them nonspecific, or have not been convincingly replicated [12] . Genome-wide association studies (GWAS) have successfully identified roughly 100 loci associated with prostate cancer risk [11] , [12] , [13] , [14] , [15] , [16] , [17] , [18] , [19] , [20] , [21] , [22] , [23] , [24] , [25] , [26] ; however, most loci have minor allele frequencies (MAFs) >10% and, so far, none conclusively differentiate aggressive from nonaggressive disease. To discover additional loci associated with risk and to identify loci specific for aggressive prostate cancer, here we conduct a multistage GWAS for prostate cancer among men of European ancestry using the Illumina HumanOmni2.5 Beadchip, which provides greater coverage of uncommon SNPs for individuals of European ancestry than microarrays used in previous GWAS of prostate cancer. We identify two novel loci associated with the Gleason score, a pathological measure of prostate cancer aggressiveness, that are located near genes involved in vascular development and maintenance. Case–control association results for prostate cancer A total of 4,600 cases and 2,941 controls of European ancestry from the Prostate, Lung, Colorectal, and Ovarian (PLCO) Cancer Screening Trial were genotyped using the Illumina HumanOmni2.5 Beadchip and passed rigorous quality-control criteria (see Methods). 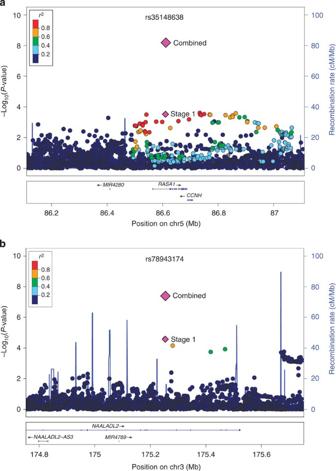Figure 1: Regional association plots of the two novel loci associated with the Gleason score as a quantitative trait among cases. (a) Chromosome 5q14.3 (rs35148638) and (b) chromosome 3q26.31 (rs78943174). Shown are the –log10associationPvalues from the linear regression model for the 4,545 cases in stage 1 (dots and lower purple diamond) and –log10Pvalues from the linear regression model for the 12,518 cases in the combined stage 1–3 analysis (upper diamond). Baseline characteristics of the cases and controls are shown in Supplementary Table 1 . On the basis of a linear regression model, men with higher Gleason scores were more likely to be diagnosed at an older age ( P <0.001). Of the SNPs genotyped, 1,531,807 passed quality-control filters with a minimum call rate of 94%. Genotypes were analysed using regression models, assuming a log-additive genetic model and adjusting for age and significant eigenvectors. A quantile–quantile (Q–Q) plot of the P values for prostate cancer risk on the basis of logistic regression models showed enrichment of small P values compared with the null distribution, even after removing SNPs within 500 kb of the previously published loci ( Supplementary Fig. 1 , λ =1.007). Fifty-six of the previously published loci were nominally associated with risk ( P <0.05) in stage 1 ( Supplementary Table 2 ), and two previously published loci at chromosomes 8q24 and 17q12 reached genome-wide significance in stage 1 ( P <5 × 10 −8 , Supplementary Fig. 2 ). Rare variant analysis using SKAT [27] for SNPs with MAF<2% revealed five gene regions with P <5 × 10 −8 ; however, all appeared to be artefacts driven by poorly clustered SNPs. Sixteen promising SNPs with P <2 × 10 −5 on the basis of the logistic regression models were taken forward for Taqman replication in 5,139 cases and 5,591 controls from seven studies (see Methods); however, none replicated for prostate cancer overall ( Supplementary Table 3 ). A more extensive replication was undertaken using a custom Illumina iSelect microarray comprising 51,207 SNPs selected for prostate cancer, 10,458 SNPs for other phenotypes (for example, obesity) and 1,435 candidate SNPs (see Methods). In stage 2, a total of 6,575 cases and 6,392 controls from five studies were genotyped with the custom iSelect and passed quality-control criteria ( Supplementary Table 1 ). In silico data were also available for stage 3 for 1,204 nonoverlapping cases and 1,231 controls from a previous GWAS of advanced (defined as Gleason score ≥8 or stage C/D) prostate cancer [12] , giving a total of 12,379 cases and 10,564 controls. As not all SNPs included on the iSelect were directly genotyped in stage 1 or stage 3, both scans were imputed using the 1000 Genomes Project release version 3 (ref. 28 ) and IMPUTE2 (ref. 29 ). In a combined meta-analysis of the primary scan together with the custom SNP microarray replication and in silico look-up in a previous GWAS, 13 loci reached genome-wide significance ( P <5 × 10 −8 ); however, each of them confirmed a previously reported locus [13] , [14] , [15] , [16] , [17] , [18] , [19] , [20] , [23] ( Supplementary Table 4 ). Although not reaching genome-wide significance, two new suggestive loci at chromosome 16q22.2 ( PKD1L3 , rs12597458, P =9.67 × 10 −8 ) and 6p22.3 ( CDKAL1 , rs12198220, P =2.13 × 10 −7 ) were also identified ( Supplementary Table 5 , Supplementary Fig. 3 ). Further studies are needed to confirm these findings. Case-only results of disease aggressiveness To evaluate disease aggressiveness, we modelled the Gleason score as a quantitative trait among the prostate cancer cases ( n =4,545) included in stage 1 in a case-only analysis using linear regression. We chose to model the Gleason score as a quantitative trait as opposed to a dichotomous outcome in order to maximize our statistical power to detect variants that differentiate aggressive from nonaggressive disease. In stage 1, the Q–Q plot of the association P values revealed a small number of SNPs with P values less than expected under the null distribution ( Supplementary Fig. 4 , λ =0.998). We evaluated the SNPs previously reported to be associated with the risk of aggressive disease; however, none were significantly associated with the Gleason score among cases ( Supplementary Table 6 ). As part of the custom SNP microarray replication, SNPs with a P value <0.001 from the linear regression model of the Gleason score as a quantitative trait, filtered using r 2 >0.8, were taken forward for the custom SNP microarray replication in 5,355 cases with the Gleason score from five studies (stage 2). One novel locus at chromosome 5q14.3 (rs35148638) reached genome-wide significance in the meta-analysis of stages 1 and 2. Five SNPs, including two moderately correlated SNPs at chromosome 5q14.3, with P values <2 × 10 −6 , were taken forward for replication in 2,618 cases from the Cancer of the Prostate in Sweden study. In the meta-analysis of the Gleason score results for all three stages including a total of 12,518 cases, three SNPs reached genome-wide significance: rs35148638 at 5q14.3 ( P =6.49 × 10 −9 ), rs62113212 at 19q13.33 ( P =5.85 × 10 −9 ) and rs78943174 at 3q26.31 ( P =4.18 × 10 −8 ; Table 1 ). The SNPs at chromosome 5q14.3 and 3q26.31 represent novel loci ( Fig. 1 ), whereas the chromosome 19q13.33 locus has been previously identified to be associated with prostate cancer risk overall [18] . Table 1 Loci associated with prostate cancer aggressiveness as measured by the Gleason score among cases only*. Full size table Figure 1: Regional association plots of the two novel loci associated with the Gleason score as a quantitative trait among cases. ( a ) Chromosome 5q14.3 (rs35148638) and ( b ) chromosome 3q26.31 (rs78943174). Shown are the –log 10 association P values from the linear regression model for the 4,545 cases in stage 1 (dots and lower purple diamond) and –log 10 P values from the linear regression model for the 12,518 cases in the combined stage 1–3 analysis (upper diamond). Full size image Stratified case–control association results for novel loci To evaluate the extent to which these three loci (identified from our case-only study of the Gleason score) could be associated with aggressive prostate cancer risk, we conducted a case–control analysis stratified by the overall Gleason score (that is, scores of 2–10), recognizing that our power to detect an association at genome-wide significance would be reduced. We did not have data on the individual components of Gleason 7 from most studies in order to subclassify them as 3+4 or 4+3, and so in order to clearly differentiate between aggressive and nonaggressive disease, we stratified our cases by those with Gleason scores ≤6 (nonaggressive) and those with Gleason ≥8 (aggressive). Although it did not reach genome-wide significance, rs35148638 at 5q14.3 showed an increased risk with aggressive prostate cancer ( P =8.85 × 10 −5 ; Supplementary Table 7 ). There was no association for nonaggressive disease ( P =0.57) and the P value for heterogeneity between the two outcomes was modestly significant ( P =2.89 × 10 −4 ). As rs78943174 at 3q26.31 was not common among controls with a MAF of 1–2%, we had limited power to detect an association with aggressive disease; however, we did observe a marginal positive association between rs78943174 and aggressive prostate cancer risk ( P =0.07) and the P value for heterogeneity between aggressive and nonaggressive prostate cancer risk was nominally significant ( P =0.006). Consistent with previous studies [30] , the SNP at 19q13.33 was strongly associated with nonaggressive prostate cancer ( P =3.51 × 10 −13 ) with a weak association in the opposite direction for aggressive prostate cancer ( P =0.01) and highly significant P value for heterogeneity ( P =1.44 × 10 −10 ). As African Americans have an elevated risk of prostate cancer, we evaluated the extent to which these three SNPs were associated with aggressive prostate cancer risk in African Americans using data from the African American Prostate Cancer GWAS Consortium (see Methods). In this smaller study, none of the SNPs were significantly associated with the risk of aggressive disease ( Supplementary Table 8 ), and only rs62113212 at chromosome 19q13.33 was nominally associated with nonaggressive disease ( P =0.04). However, the direction of the effects for African Americans for the SNPs at 3q26.31 and 19q13.33 were consistent with what we observed among Europeans. Further examination of novel loci Examination of the three identified loci for the Gleason score using data from ENCODE revealed significant DNase enrichment in lymphoblastoid and embryonic myoblast cells and evidence for altered motifs ( Supplementary Table 9 ). Rs62113212 at 19q13.33 is in strong linkage disequilibrium with a missense SNP (rs17632542, r 2 =1). No significant expression quantitative trait locus (eQTL) associations were observed using data from the Genotype-Tissue Expression (GTEx) Project [31] ; however, for a proxy of rs35148638 at 5q14.3 (rs4421140, r 2 =0.82), we did find nominally significant eqtl associations with RASA1 and CCNH expression and meqtl associations with CpG sites in RASA1 and CCNH in adipose tissue [32] , [33] . Linkage studies of prostate cancer aggressiveness have reported suggestive evidence of linkage to chromosome 5q (refs 5 , 6 , 7 , 8 ) and specifically 5q14 in TMPRSS2-ERG fusion-positive families [34] . The 5q14.3 SNP identified in this study (rs35148638), associated with disease aggressiveness, is intronic to the RAS p21 protein activator 1 ( RASA1 ) gene, which suppresses RAS function, helps regulate cellular proliferation and differentiation [35] , and controls blood vessel growth [36] . Rare mutations in RASA1 lead to capillary malformation-arteriovenous malformation and Parkes–Weber syndrome [37] as well as lymphatic abnormalities [38] , providing an intriguing plausibility for the gene in aggressive prostate cancer. The SNP is also ∼ 79 kb downstream of the cyclin H ( CCNH ) gene, which encodes a regulatory component of a cyclin-dependent (CDK)-activating kinase necessary for RNA polymerase II transcription, nucleotide excision repair and p53 phosphorylation [39] . CCNH has been shown to be differentially expressed between androgen-sensitive and androgen-resistant prostate cancer cell lines [40] , [41] , suggesting a role in prostate cancer progression. The 3q26.31 SNP (rs78943174) is intronic to the N-acetylated alpha-linked acidic dipeptidase-like2 ( NAALADL2 ) gene, which is part of the glutamate carboxypeptidase II family. This gene is also related to prostate-specific membrane antigen, a well-characterized diagnostic indicator and potential drug target of prostate cancer [42] . NAALADL2 has been shown to promote a pro-migratory and pro-metastatic microenvironment, and higher tumour expression of NAALAD2 is associated with higher Gleason score and poor survival following radical prostatectomy [43] . Variants in NAALADL2 have also been identified to be associated with Kawasaki disease [44] , a paediatric, autoimmune vascular disease. The SNP is also ∼ 117 kb telomeric of the microRNA, MIR4789, which is predicted to target several genes involved in the insulin resistance (for example, IRS1, PIK3R1 ) among others [45] , [46] . A previous GWAS of prostate cancer reported a suggestive association with a SNP at 3q26.31 (ref. 47 ); however, this SNP is not in linkage disequilibrium with the SNP identified in our study ( r 2 =0.003). The chromosome 19q13.33 ( KLK3 ) locus has been previously associated with prostate cancer risk overall [18] . Although several studies have suggested that the risk may differ by disease aggressiveness [30] , [48] , [49] , [50] , this study shows for the first time a genome-wide significant difference between aggressive and nonaggressive disease as measured by the Gleason score. KLK3 encodes the prostate-specific antigen (PSA) protein. The C allele of rs62113212 has been shown to be associated with higher PSA levels [48] , suggesting that the association observed with the SNP is related to early prostate cancer detection. Although one of our goals was to identify uncommon variants for prostate cancer, we did not identify any new independent SNPs with a MAF <10%. We did, however, identify a suggestive locus at chromosome 6p22.3 (rs12198220), which is 98 kb downstream of CDKAL1 , A pooled linkage study of prostate cancer previously reported suggestive evidence of linkage to this region [51] . Interestingly, SNPs at this locus have been associated with the risk of type 2 diabetes, adding to the list of susceptibility regions shared between prostate cancer and type 2 diabetes [52] . We also discovered a new suggestive locus at 16q22.2, which is in strong linkage disequilibrium with a missense variant (rs3213422, r 2 =0.74) in dihydro-orotate dehydrogenase (quinone) gene ( DHODH ), which encodes an enzyme necessary for the biosynthesis of pyrimidines and cell proliferation. Further studies are needed to confirm these suggestive loci. In this study, we used the Gleason score to differentiate between nonaggressive and aggressive prostate cancer. Gleason score is a powerful prognostic factor and predictor of disease behaviour; however, substantial changes in Gleason scoring have changed since it was first proposed over 40 years ago, resulting in shifts towards higher scores [53] . In addition, differences in scoring between pathologists remain [54] . Whether these changes in Gleason scoring ultimately result in better outcome prediction and classification of disease from an aetiologic standpoint remains to be seen. Unlike for breast cancer where classification by receptor status has resulted in significant advances in the aetiologic understanding of the disease, clearly defining aggressive prostate cancer remains difficult. Regardless, the Gleason score is an important component of prostate cancer risk assessment and is the most commonly used tool for assessing prostate cancer aggressiveness. In conclusion, we identified two new loci associated with prostate cancer aggressiveness as measured by the Gleason score in a case-only study of prostate cancer. Although additional studies are needed to confirm these findings and reveal the underlying biological mechanism, the proximity of these SNPs to genes involved in vascular disease, cell migration and metastasis makes them intriguing loci for further study. Stage 1: discovery population and genotyping A new GWAS was conducted in prostate cancer cases and controls of European ancestry from the PLCO Cancer Screening Trial. PLCO is a randomized trial for the early detection of prostate, lung, colorectal and ovarian cancers [55] . In brief, 76,693 men were enrolled in the trial from 10 centres in the United States from 1993 to 2001 and randomized to receive annual screening with PSA for 6 years and digital rectal examination for 4 years or referred to their physician for routine care. Men with positive screening results were referred to their primary physician for further evaluation. All prostate cancer cases detected during screening or reported during the trial were pathologically confirmed, and information on stage and grade was abstracted from medical records. Blood or buccal cells were collected from participants in the trial [56] . The study was approved by the institutional review board at each centre and National Cancer Institute (NCI); all study participants provided informed written consent. A total of 4,838 prostate cancer cases and 3,053 controls of European ancestry, matched on age and year of randomization, were selected for stage 1. The sample size was chosen on the basis of statistical power estimates for detecting a modest association in a multistage GWAS. Including quality-control duplicates, 8,222 samples were genotyped on the Illumina HumanOmni2.5 Beadchip. Extensive quality-control metrics were employed to ensure that only high-quality genotype data were analysed using the GLU software package. Samples with a missing rate >6% ( n =323) or heterozygosity <16% or >21% ( n =7) were excluded, and 221 samples were removed because of technical issues. Gender discordance on the basis of chromosome X heterozygosity was evaluated; however, no subjects were removed. One unexpected duplicate (>99.9% concordance) and 28 full sibling pairs on the basis of an identity-by-descent threshold of 0.70 were detected and one subject from each pair was removed ( n =29). Ancestry was estimated using a set of population informative markers [57] and the GLU struct.admix module, which is similar to the method proposed in (ref. 58 ). Five subjects (three cases and two controls) were determined to have <80% European ancestry and were removed from analysis ( Supplementary Fig. 5 ). Principal components analysis was performed to evaluate population substructure in greater detail ( Supplementary Fig. 6 ), and two significant eigenvectors ( P <0.05) were included in the analytic model. Expected duplicates yielded 99.9% concordance. SNPs without genotype calls, a completion rate <94%, Hardy–Weinberg proportion test P value <1 × 10 −8 or MAF<1% were excluded, leaving 1,531,807 SNPs for analysis. After quality-control exclusions, 4,600 cases and 2,840 controls remained. An additional 101 male controls from PLCO Cancer Screening Trial, genotyped previously on the HumanOmni2.5 (ref. 59 ) were also included, resulting in 4,600 cases and 2,941 controls for the primary prostate cancer analysis ( Supplementary Table 1 and Supplementary Fig. 7 ). Of those cases, 4,545 men had information on the Gleason score available. Regression models were fit adjusting for significant principal components and age. Sixteen different models were fitted for prostate cancer-related outcomes, including overall prostate cancer risk and Gleason score. Stage 2: follow-up studies and genotyping Replication was conducted using a set of independent prostate cancer cases and controls from five studies: Alpha-Tocopherol, Beta-Carotene Cancer Prevention Study [60] (ATBC, n =1,092 cases/1,099 controls), Cancer Prevention Study II (ref. 61 ; CPSII, n =2,770 cases/2,669 controls), Health Professional Follow-up Study [62] ( n =963 cases/1,047 controls), French Prostate Cancer Case–Control Study ( n =1,494 cases/1,546 controls) and PLCO [55] ( n =990 cases/922 controls). Including quality-control duplicates, 14,592 samples were genotyped using a custom Illumina iSelect microarray comprising 51,207 SNPs selected for prostate cancer, 10,458 SNPs for other phenotypes (for example, smoking and obesity) and 1,435 candidate SNPs. The SNPs for prostate cancer were filtered using r 2 <0.7 and selected on the basis of the most significant results from 16 prostate cancer models, with the primary models being an overall prostate cancer risk model assuming a log-additive effect for each SNP and case-only Gleason score model, where Gleason was modelled as a quantitative linear trait among cases and each SNP was assumed to have an additive effect. SNPs with P values <0.05 and <0.001 from each model, respectively, were advanced for possible replication. Similar to stage 1, samples genotyped in stage 2 underwent rigorous quality-control procedures. Samples with missing rate >10% ( n =1,158) or mean heterozygosity <20% or >26% ( n =4) were excluded. In addition, 21 subjects without phenotype information were removed. Fifteen unexpected duplicates with concordance rates >99.9% were observed, and 25 first-degree relative pairs were detected assuming an identity-by-descent threshold of 0.7. For each unexpected duplicate and relative pair, one subject was removed. Using the GLU struct.admix module, ancestry was estimated on the basis of genotyped SNPs with a MAF>10% and HapMap data as the fixed reference population. Sixty-six subjects with <80% European ancestry were removed from the analysis. Principal components analysis was conducted using a set of SNPs selected for traits unrelated to prostate cancer (for example, smoking and alcohol intake). After quality-control exclusions, a total of 6,575 cases and 6,392 controls remained for the primary analysis ( Supplementary Table 1 ), including 5,355 cases with the Gleason score. SNPs with a MAF<1% or completion rate <90% were excluded from the analysis, leaving 55,497 SNPs for analysis ( Supplementary Fig. 7 ). Regression models were fit adjusting for age, significant principal components and study. In addition to the custom SNP microarray replication, 16 promising SNPs ( P <2 × 10 −5 ) were taken forward for fast-track replication in the five studies listed above ( n =2,495 cases/2,532 controls) as well as three additional studies: Agricultural Health Study [63] ( n =579 cases/1,172 controls), Fred Hutchinson Cancer Research Center ( n =1,315 cases/1,152 controls) and the Multiethnic Cohort [64] ( n =750 cases/735 controls). In total, 5,139 cases and 5,591 controls, all of European ancestry, were genotyped ( Supplementary Fig. 7 ). The SNPs were genotyped using individual TaqMan assays (Applied Biosystems Inc) and quality-control duplicates yielded >99.9% concordance. Stage 3a: in silico replication of prostate cancer findings For replication of the overall prostate cancer results, nonoverlapping in silico GWAS data were available from 1,204 cases and 1,231 controls of European ancestry from four studies from a previous GWAS of advanced prostate cancer [12] : European Prospective Investigation into Cancer and Nutrition (EPIC; 431 cases/426 controls) [65] , Multiethnic Cohort (244 cases/259 controls) [64] , Physicians Health Study (PHS; 298 cases/255 controls) and American Cancer Society Cancer Prevention Study II (CPSII; 231 cases/291 controls not included in stage 2) [61] ( Supplementary Fig. 7 ). Subjects were genotyped using the Illumina HumanHap610K and extensive quality-control filters applied as described previously. All data were imputed using IMPUTE2 (ref. 29 ) and 1000 Genomes Project release version 3 (ref. 28 ) as the reference panel, and data analysed using SNPTEST assuming a log-additive genetic model and adjusting for age, study and significant principal components. Only SNPs with an information score >0.3 were included in the meta-analysis. Stage 3b: additional replication for Gleason score findings For further replication of the results for the Gleason score, we genotyped five of the most significant SNPs ( P <2 × 10 −6 ) in the Cancer of the Prostate in Sweden, a population-based case–control study of 2,618 cases and 1,728 controls using Sequenom ( Supplementary Fig. 7 ). Regression models were fit adjusting for age. Meta-analysis Data from all three stages were meta-analysed using the fixed effects inverse variance method based on the beta estimates and s.e.’s from each stage. Further follow-up analyses To evaluate the associations observed in our study of men of European ancestry with those observed in African Americans, we obtained association results for three genome-wide significant hits from the African American Prostate Cancer GWAS Consortium [22] . Although it was not possible to evaluate the Gleason score as a quantitative trait among cases in this consortium, we were able to obtain stratified association results for cases with Gleason ≤6 versus controls and cases with Gleason ≥8 versus controls. Using 1000 Genomes Project data, we identified SNPs with r 2 >0.8 with the lead SNPs identified to be associated with Gleason score and evaluated whether they were nonsynonymous coding variants. We utilized HaploReg [66] to assess noncoding functional markers in the regions containing our lead SNPs and related proxy SNPs ( r 2 >0.8; Supplementary Table 9 ). We explored possible cis eQTL associations with our lead SNPs and related proxy SNPs ( r 2 >0.8) in adipose tissue, lymphoblastoid cell lines and skin using data from the MuTHER resource [32] and all available tissues, including whole blood, in the GTEx [31] . We also examined possible methylation eQTL associations in adipose tissue using the MuTHER resource [33] . Accession number: The GWAS data from stage 1 is available on dbGaP under accession number phs000882.v1.p1. How to cite this article : Berndt, S. I. et al , Two Susceptibility Loci Identified for Prostate Cancer Aggressiveness. Nat. Commun , 6:6889 doi: 10.1038/ncomms7889 (2015).